Inertio-elastic focusing of bioparticles in microchannels at high throughput Controlled manipulation of particles from very large volumes of fluid at high throughput is critical for many biomedical, environmental and industrial applications. One promising approach is to use microfluidic technologies that rely on fluid inertia or elasticity to drive lateral migration of particles to stable equilibrium positions in a microchannel. Here, we report on a hydrodynamic approach that enables deterministic focusing of beads, mammalian cells and anisotropic hydrogel particles in a microchannel at extremely high flow rates. We show that on addition of micromolar concentrations of hyaluronic acid, the resulting fluid viscoelasticity can be used to control the focal position of particles at Reynolds numbers up to Re ≈10,000 with corresponding flow rates and particle velocities up to 50 ml min −1 and 130 m s −1 . This study explores a previously unattained regime of inertio-elastic fluid flow and demonstrates bioparticle focusing at flow rates that are the highest yet achieved. The ability to continuously manipulate and separate particles or cells from very large volumes of fluids at high throughput is critical for many biomedical, environmental and industrial applications [1] , [2] . Although microfluidic technologies such as immunoaffinity capture [3] , deterministic lateral displacement [4] and microporous filtration [5] have revolutionized the sorting of cells from bodily fluids, they have typically been limited to low throughput. More recently, directed inertial migration of particles toward specific fluid streamlines (initially observed in centimeter-scale pipe flows [6] ) has been observed in straight [7] , [8] and curved [9] , [10] microchannels in Newtonian fluids (of density ρ and constant shear viscosity ) at moderate Reynolds numbers ( Re = ρUH /η≈100), where U is the particle velocity and H is the channel cross-sectional dimension. However, the upper bound of sample throughput for inertial focusing in a straight microchannel is limited by the hydrodynamic transition from laminar flow to turbulent flow and has only been observed for Re ≤1,500 (ref. 11 ), and in curved channels it is limited by dominant Dean drag forces relative to inertial lift forces [12] . In separate studies, particle migration due to elastic effects has also been explored [13] , [14] using particles suspended in viscoelastic fluids at moderate to high Weissenberg numbers [15] ( Wi = λU / H , where λ is the characteristic relaxation time), but here controlled viscoelastic focusing was limited to only low Reynolds numbers ( Re <<1). Recently, particle migration toward the centerline of a microchannel has been observed in a viscoelastic fluid with non-negligible inertial effects; however, particle focusing destabilized as the channel Reynolds number increased beyond order unity [16] , [17] . Fluid inertia and fluid elasticity are both nonlinear effects that tend to destabilize a flow when acting alone [18] , [19] , but if they are simultaneously present, then they can interact constructively to stabilize a given flow [20] , [21] . However, at present, it is unknown whether weakly viscoelastic flows at high Reynolds number ( Re >2,000) can facilitate inertio-elastic particle migration in microchannels. There are significant technical challenges to studying particle focusing at very high Reynolds numbers. One challenge is building microfluidic devices that can withstand pressure drops that may easily approach 5,000 psi (3.4 × 10 7 Pa) depending on channel dimensions and operating flow rate. Another challenge is tracking individual particles with particle velocities that can easily exceed 100 m s −1 . Here, we show that on the addition of micromolar concentrations of hyaluronic acid (HA), the resulting fluid viscoelasticity can be used to control the focal position of bioparticles at Reynolds numbers up to Re ≈10,000 in a rigid (epoxy-based) microchannel. This corresponds to flow rates and particle velocities up to 50 ml min −1 and 130 m s −1 . We find that it is not secondary flows or shear thinning in the fluid rheology but rather the presence of viscoelastic normal stresses that drive the deterministic particle migration in the HA solution. Furthermore, the rheological properties of the viscoelastic fluid can be tuned to generate an optimal balance between particle focusing and particle stretching in mammalian cells over a wide range of Reynolds numbers. Our results demonstrate that particle focusing in an unexplored fluid regime occurs in a manner that appears distinct relative to previously observed modes of particle focusing. We anticipate this study to motivate the development of microfluidic technologies capable of high-throughput particle sorting from very large fluid volumes. Flow regime characterization Here, we used an epoxy-based fabrication technique ( Supplementary Fig. 1 ) to construct a 35-mm long straight channel with H =80±5 μm square cross-section capable of achieving a maximum throughput of Q =50 ml min −1 ( Re =10,400, U =130 m s −1 ). We infused test fluids into the microchannel using a high-pressure (up to 10,000 psi), high-throughput (up to 50 ml min −1 ) syringe pump. Long-exposure fluorescence (LEF) imaging was used to efficiently detect particle migration based on aggregate signal intensity ( Fig. 1a ). Particle trajectory analysis [22] was used to observe specific features (for example, 3D position, orientation, deformation) of the particle migration based on individual particle statistics. Microparticle imaging velocimetry (μ-PIV) was used to measure the local fluid velocity in the microchannel (based on 1-μm polystyrene beads), while particle tracking velocimetry (PTV) was used to measure discrete particle velocities in the microchannel (based on 8-μm polystyrene beads). 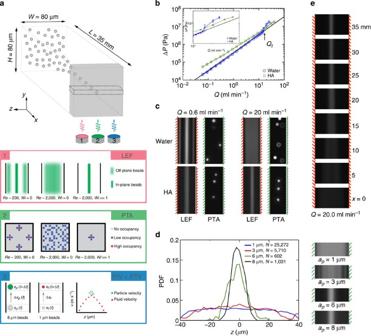Figure 1: Particle focusing at high flow rates in water and HA solutions. (a) Imaging techniques used to observe 8-μm particles (particle velocity and position) and 1-μm particles (fluid velocity). (b) Pressure drop across the fluidic system. The solid grey line indicates the expected pressure drop for the laminar flow of water in the microchannel. Inset plot shows pressure drops near the onset of inertially turbulent flow atQ=Qt. (c) LEF provides average particle distribution based on mean fluorescence intensity. Particle trajectory analysis provides two-dimensional particle histogram based on in-focus particles at a given imaging plane. The hashed lines indicate location of the rigid channel walls. A flow rate ofQ=0.6 ml min−1corresponds toRe=140 in water, and toRe=105 andWi=17 in the viscoelastic HA solution. A flow rate ofQ=20.0 ml min−1, corresponds toRe=4,630 in water andRe=4,422 andWi=566 in HA. (d) Probability density function determined fromNparticles sized fromap=1, 3, 6 and 8 μm (volume fractionϕ=2.0% for 1 μm andϕ=0.05% for 3, 6 and 8 μm) across the channel width determined from short-exposure images with pulsed laser illumination. The corresponding LEF images are shown adjacent to the plot. (e) LEF images of 8-μm particles at 5-mm intervals along the length of the channel atQ=20 ml min−1, showing the lateral migration of the particles towards the centerline. Figure 1: Particle focusing at high flow rates in water and HA solutions. ( a ) Imaging techniques used to observe 8-μm particles (particle velocity and position) and 1-μm particles (fluid velocity). ( b ) Pressure drop across the fluidic system. The solid grey line indicates the expected pressure drop for the laminar flow of water in the microchannel. Inset plot shows pressure drops near the onset of inertially turbulent flow at Q = Q t . ( c ) LEF provides average particle distribution based on mean fluorescence intensity. Particle trajectory analysis provides two-dimensional particle histogram based on in-focus particles at a given imaging plane. The hashed lines indicate location of the rigid channel walls. A flow rate of Q =0.6 ml min −1 corresponds to Re =140 in water, and to Re =105 and Wi =17 in the viscoelastic HA solution. A flow rate of Q =20.0 ml min −1 , corresponds to Re =4,630 in water and Re =4,422 and Wi =566 in HA. ( d ) Probability density function determined from N particles sized from a p =1, 3, 6 and 8 μm (volume fraction ϕ =2.0% for 1 μm and ϕ =0.05% for 3, 6 and 8 μm) across the channel width determined from short-exposure images with pulsed laser illumination. The corresponding LEF images are shown adjacent to the plot. ( e ) LEF images of 8-μm particles at 5-mm intervals along the length of the channel at Q =20 ml min −1 , showing the lateral migration of the particles towards the centerline. Full size image To study particle migration in viscoelastic flows at high Reynolds number, we selected HA as a model viscoelastic additive based on its biocompatibility and the turbulent drag-reducing properties that have been documented in the flow of blood [23] and synovial fluid [24] . The Reynolds number was calculated based on a shear rate-dependent viscosity as defined by the Carreau model ( Supplementary Fig. 2 ). This viscosity is evaluated at the relevant wall shear rate in the fluid given by , based on the analytical solution for the velocity field of a Newtonian liquid in a square channel (with cross-sectional dimension H ). The Weissenberg number was calculated based on a fluid relaxation time λ =8.7 × 10 −4 s measured experimentally using the thinning dynamics of a liquid filament [25] . The measured pressure drop Δ P over the entire fluidic network was measured by the syringe pump for a given imposed flow rate Q ( Fig. 1b ). For water, Δ P water first increased linearly with Q before increasing more rapidly at Re ≈2,500±500, which indicated a transition to turbulence. In the HA solution, Δ P HA scaled sublinearly with Q due to shear thinning effects, and Δ P HA >Δ P water (due to the higher fluid viscosity) for Q < Q t , where Q t ≈12±2.5 ml min −1 is the flow rate at which the flow of water transitioned from laminar to turbulent. However, for flow rates Q > Q t , Δ P HA continued to scale sublinearly with Q (up to 50 ml min −1 ), which suggests that the flow of the HA solution remained laminar even up to Re ≈10,000. Using a microfluidic rheometer we also measured the viscosity of the HA solution ( M w =1,650 kDa, 0.1% w/v) before and after sample processing within the range of shear rates explored in the microchannel . Over this range of shear rates the shear viscosities of the native and used samples were found to remain almost unchanged, indicating that shear-induced degradation of the sample [26] was not a major issue ( Supplementary Fig. 2 ). Particle focusing characterization With the ability to achieve laminar microchannel flow at a Reynolds number up to Re ≈10,000 in a viscoelastic HA solution, we focused our attention on the importance of persistent laminar flow conditions on inertio-elastic particle focusing. We first observed the flow behaviour of 8-μm beads in HA for Q < Q t . At Q =0.6 ml min −1 ( Re =105, Wi =17), we observed particle migration towards a single centralized point along the channel centerline ( Fig. 1c ). This focusing behaviour was also observed at flow rates as high as Q =6 ml min −1 ( Supplementary Fig. 3 , Re =1,270, Wi =170). The results obtained in the viscoelastic HA solution were in stark contrast to those in a Newtonian fluid. In water, beads initially focused to four off-centre equilibrium positions near each face of the rectangular microchannel at Q =0.6 ml min −1 ( Re =140) before shifting to a five-point quincunx configuration at Q =6 ml min −1 ( Re =1,400) with equilibrium positions at the centerline and the four channel corners, where the shear rate is lowest. These experimental observations in water were in broad agreement with previous numerical studies of inertial migration in Newtonian fluids [27] , [28] . Having established that particle focusing can be achieved for Q < Q t in both water and HA solution, albeit with significant configurational differences, we set Q > Q t to determine if deterministic particle focusing could be preserved in either fluid. For Q >13 ml min −1 in water ( Re >2,000), particle tracking showed that the fluorescent beads were randomly distributed throughout the channel due to the onset of inertial turbulence, and this critical flow rate corresponded closely to the critical conditions beyond which Δ P water increased superlinearly with increasing Q . Surprisingly, for Q > Q t , beads in the HA solution continued to focus towards a centralized point along the channel centerline and we found that particle focusing in the HA solution persisted to Reynolds numbers well above the upper limit that could be attained for particle focusing in water. These results represent the highest flow rates at which deterministic particle focusing has been achieved in a microchannel and illustrate the precise focusing control that can be achieved by using only small amounts of a viscoelastic drag-reducing polymeric agent (HA). Given the well-known dependence of focusing efficiency on particle diameter a p for inertial focusing [12] , [29] , and creeping flows of viscoelastic fluids [30] , we studied the effect of particle size on the inertio-elastic particle focusing observed in the HA solution. Using polystyrene beads with a p =1, 3, 6 or 8 μm, we found that particle focusing toward the channel centre in HA solution improved with increasing particle size at Q =20 ml min −1 ( Fig. 1d , Re =4,422, Wi =566). Theoretical analysis of a single particle in the creeping flow limit [31] shows that the elastic lift force on a spherical particle in a weakly elastic fluid undergoing a pressure-driven shear flow scales as F L,E ~2 ηλU 2 ( a p / H ) 3 ( Supplementary Note 1 ). In contrast, the lateral resistive Stokes drag that resists particle migration only scales linearly with particle size a p and with the migration velocity u mig . Hence, the value of u mig is expected to scale strongly with a p , meaning that a larger particle should require a much shorter distance to reach its equilibrium position. Using LEF images captured along the entire length of the microchannel at Q =20 ml min −1 ( Fig. 1e ), we found that 8-μm beads laterally migrated to their equilibrium position within an equilibrium focusing length L f ≤30 mm, based on the invariant width of the focused streak further downstream ( Supplementary Fig. 4 ). In contrast, at the same flow rate, lateral migration of 6-μm beads was incomplete within the channel length L =35 mm. In order to provide further insight into the physical basis of inertio-elastic particle focusing in the HA solution, we carried out a comparative study of water and HA solution within the laminar regime. For a given flow rate, we constructed vector plots of fluid velocity ( Fig. 2a ) based on 1-μm neutrally-buoyant beads being convected with the fluid through the microchannel, and also constructed ‘heat maps’ of particle occurrence frequency across the channel cross-section based on the two-dimensional position of 8-μm beads moving through the microchannel ( Fig. 2b ). We then combined the velocity profiles with the individual particle statistics ( Fig. 2c ). We first considered the effect of shear thinning on particle focusing in HA solution. This was motivated by previous work [13] suggesting that shear thinning in the fluid viscosity drives particles toward the wall. At Q =0.09 ml min −1 , we observed a markedly more blunt fluid velocity profile in the HA solution compared with water ( Fig. 2c ), which is consistent with the shear thinning behaviour observed at ( Supplementary Fig. 2 ) and with computational simulations using the Carreau model. At Q =6 ml min −1 , the characteristic shear rate in the fluid increased to where the viscosity varied less strongly with shear rate. We continued to observe particle focusing towards the centre in the HA solution despite nearly identical fluid velocity profiles (measured using μ-PIV with 1-μm beads) for water and the HA solution ( Fig. 2c ). This result suggests that shear thinning in the velocity profile did not play a dominant role in particle focusing under these flow conditions. 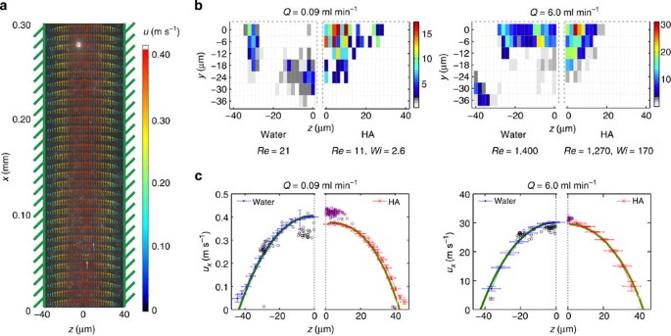Figure 2: Features of inertio-elastic focusing based on individual particles. (a) Representative fluid velocity field along the channel determined from a correlative μ-PIV technique. (b) Cross-sectional particle histogram of 8-μm particles in a lower quadrant of the square cross-section channel atQ=0.09 ml min−1and atQ=6.0 ml min−1. (c) Velocity profiles measured in the two fluids (red and blue curves respectively) and the corresponding velocities of the migrating 8-μm beads (black dots for beads in water and violet dots for beads in the HA solution) measured at the channel mid-plane (y=0 μm). Note that atQ=0.09 ml min−1in water, the particles occupy off-center equilibrium positions with fourfold symmetry. The particles that appear to be located atz=0 inFig. 2care projections of particles located aroundy≈±25 μm. For comparison, the expected velocity profiles at the mid-plane of the channel (that is,y=0 μm) for the flow of a Newtonian fluid and a shear thinning Carreau model (determined from COMSOL simulations) are shown by the green and gold curves, respectively. The s.d. in the velocity measurements are shown by the error bars inux, and the width of the interrogation windows are shown by the error bars along thez-axis. Figure 2: Features of inertio-elastic focusing based on individual particles. ( a ) Representative fluid velocity field along the channel determined from a correlative μ-PIV technique. ( b ) Cross-sectional particle histogram of 8-μm particles in a lower quadrant of the square cross-section channel at Q =0.09 ml min −1 and at Q =6.0 ml min −1 . ( c ) Velocity profiles measured in the two fluids (red and blue curves respectively) and the corresponding velocities of the migrating 8-μm beads (black dots for beads in water and violet dots for beads in the HA solution) measured at the channel mid-plane ( y =0 μm). Note that at Q =0.09 ml min −1 in water, the particles occupy off-center equilibrium positions with fourfold symmetry. The particles that appear to be located at z =0 in Fig. 2c are projections of particles located around y ≈±25 μm. For comparison, the expected velocity profiles at the mid-plane of the channel (that is, y =0 μm) for the flow of a Newtonian fluid and a shear thinning Carreau model (determined from COMSOL simulations) are shown by the green and gold curves, respectively. The s.d. in the velocity measurements are shown by the error bars in u x , and the width of the interrogation windows are shown by the error bars along the z -axis. Full size image One important difference between the measured velocity profiles in water and the HA solution is the relationship between the average fluid velocity u f and the corresponding particle velocity u p once the focusing has fully developed (that is, x > L f ; Fig. 2c ). At each flow rate, the measured centerline velocity of the 8-μm beads in the HA solution was found to be faster than the local fluid velocity. For example, at Q =6.0 ml min −1 , the measured velocity of the beads was u p =30.9±0.7 m s −1 in the HA solution compared with a local fluid velocity of u f =30.2 m s −1 ( Fig. 2c ). In contrast, in water, the particles along the centerline translated at u p =28.2±0.9 m s −1 , which was slower than the local fluid velocity. These trends are consistent with (i) a drag increase expected for a sphere moving in a Newtonian channel flow, given by Faxén’s law for creeping flow and an Oseen correction for fluid inertia [32] , [33] , as well as (ii) the viscoelastic drag decrease on a sphere that is initially expected at a moderate particle Weissenberg number [34] , [35] . We also considered the effect of secondary flows on particle focusing in HA solution ( Supplementary Note 2 ). This was motivated by recent work [36] , [37] , [38] showing that in channels with non-axisymmetric cross-section, normal stress differences in a viscoelastic fluid can drive secondary recirculating flows that are superposed on top of the primary axial flow field. Comparing the migration behaviour of 8-μm beads in a 50-μm square (non-axisymmetric) channel and in a corresponding cylindrical (axisymmetric) tube, we observed particle focusing toward the centerline in both cases. Gaussian fits to the LEF intensity profiles observed at x > L f were indistinguishable to within one particle diameter ( Supplementary Fig. 5 ), indicating that secondary flows did not play a significant role. Bioparticle focusing in microchannels We then considered the effect of viscoelastic normal stress differences on particle focusing in HA solutions. Early theoretical work in the creeping flow limit [31] has shown that particle migration in the direction of minimum shear rate (that is, towards the channel centerline) is induced by gradients in the normal stress differences that are present when the shear rate in the fluid varies transversely in the undisturbed flow field around the particle. Numerical simulations of particle sedimentation in quiescent viscoelastic fluids have also demonstrated that viscoelastic stresses drive particles towards the centerline of channels and tubes [39] , [40] , and μ-PIV experiments have shown that fluid viscoelasticity can dramatically change the local velocity field around a particle near a wall [41] . Fully developed numerical simulations of inertio-elastic particle migration are only just beginning to become feasible (and are presently limited to moderate Weissenberg numbers ( Wi <50) and Reynolds numbers ( Re <40) [42] ) but having eliminated shear thinning and secondary flows as primary drivers of this centerline focusing it is clear that the role of viscoelastic normal stresses cannot be neglected. We used the deformability of human white blood cells (WBCs) to directly visualize the effects of normal stress differences in the fluid, which create an additional tensile stress along streamlines [15] . Because of the high spatial fidelity and lack of particle blurring afforded by the short duration of the pulsed laser imaging (δ t =10 ns), we are able to quantify the distortional effects of this streamline tension on the shape of an individual particle up to shear rates . The magnitude of WBC deformation was expressed in terms of a mean aspect ratio AR = a x / a z ( Fig. 3a ). For WBCs suspended in phosphate-buffered saline (PBS), the aspect ratio monotonically increased from AR =1.0 (at Q =0.6 ml min −1 , Re =140) to AR =1.2 (at Q =13 ml min −1 , Re =3,033) due to the increasing variation in the magnitude of the viscous shear stress acting across the WBC. In contrast, for WBCs suspended in the 1,650 kDa HA solution, the aspect ratio monotonically increased from AR =1.4 (at Q =0.6 ml min −1 , Wi =17, Re =105) to AR =2.5 (at Q =13 ml min −1 , Wi =368, Re =2,840). However, we observed a breakdown in the focusing of these deformable particles in both fluids at higher flow rates. For WBCs in a Newtonian fluid, the focusing behaviour was lost due to onset of turbulence for Q > Q t . In contrast, the focusing capacity of WBCs in a viscoelastic fluid appeared to diminish due to a combination of excessive cell stretching and the corresponding reduction in the hydraulic diameter of the cells ( Fig. 3b ). 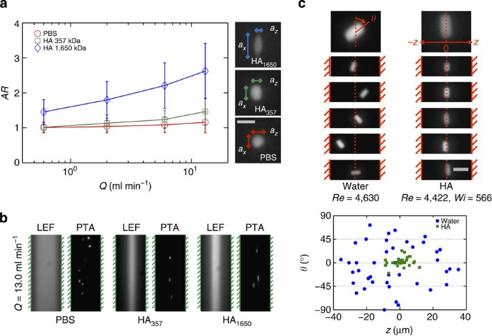Figure 3: Inertio-elastic focusing of bioparticles based on deformability and shape. (a) Deformation statistics of WBCs in PBS, a low-molecular weight (357 kDa) HA solution and a high-molecular weight (1,650 kDa) HA solution. The magnitude of WBC stretching is expressed in terms of aspect ratioAR=ax/az. Scale bar, 10 μm. The error bars indicate the s.d. in the WBC aspect ratio at each flow rate. (b) LEF and particle trajectory analysis images of WBCs in PBS, 357 kDa HA solution and 1,650 kDa HA solution atQ=13 ml min−1. (c) Particle trajectory analysis (PTA) images of anisotropic PEG particles in 1,650 kDa HA solution atQ=20 ml min−1. Dashed red lines indicate channel centerline. Scale bar, 30 μm. Measurements of lateral positionzand instantaneous orientation angleθare plotted for each PEG particle in water (blue) and in the HA solution (green). Figure 3: Inertio-elastic focusing of bioparticles based on deformability and shape. ( a ) Deformation statistics of WBCs in PBS, a low-molecular weight (357 kDa) HA solution and a high-molecular weight (1,650 kDa) HA solution. The magnitude of WBC stretching is expressed in terms of aspect ratio AR = a x / a z . Scale bar, 10 μm. The error bars indicate the s.d. in the WBC aspect ratio at each flow rate. ( b ) LEF and particle trajectory analysis images of WBCs in PBS, 357 kDa HA solution and 1,650 kDa HA solution at Q =13 ml min −1 . ( c ) Particle trajectory analysis (PTA) images of anisotropic PEG particles in 1,650 kDa HA solution at Q =20 ml min −1 . Dashed red lines indicate channel centerline. Scale bar, 30 μm. Measurements of lateral position z and instantaneous orientation angle θ are plotted for each PEG particle in water (blue) and in the HA solution (green). Full size image We have also investigated the role of fluid rheology in manipulating the interplay of particle focusing and particle stretching. In order to reduce the magnitude of the viscoelastic normal stresses experienced by WBCs, we used a lower molecular weight (357 kDa) HA solution. From the Zimm scaling for dilute polymer solutions ( λ ~ M w 0.8 ), we can estimate the relaxation time for this less viscoelastic solution to be λ 357 kDa ≈2.6 × 10 −4 s, and the Weissenberg number is reduced to Wi ≈100 at Q =13 ml min −1 . Pulsed laser images indicate the maximum anisotropy in the cell dimensions was reduced to AR =1.4 and we observed enhanced WBC focusing at flow rates beyond Q =13 ml min −1 . These results suggest that by tuning the nonlinear rheological properties of the viscoelastic working fluid it is possible to control both particle focusing and particle deformation. Recent work [43] , [44] has suggested that inertial focusing of non-spherical particles depends on the rotational diameter of a particle, regardless of its cross-sectional shape. Microscopic video imaging also shows that these particles rotate freely when suspended in a Newtonian fluid. To investigate the effect of particle shape on inertio-elastic focusing in HA solution at high Reynolds numbers, we used cylindrical cross-linked poly(ethylene glycol) (PEG) particles synthesized via flow lithography [45] . For a given PEG particle, we measured the lateral position z p (with channel centerline defined by z =0 μm) and the instantaneous orientation angle θ p of the particle (with streamwise alignment defined by θ =0°) in the original HA solution at Q =20 ml min −1 ( Fig. 3c ) poly (ethylene glycol). PEG particles in water occupied the entire range of lateral positions (−40 ≤z ≤40 μm) and orientations (−90°≤ θ ≤90°). In contrast, in the HA solution, the PEG particles exhibited strong streamwise alignment along the channel centerline with z p →0 and θ p →0. Similar streamwise alignment and migration to the centerline has been predicted in numerical simulations of the sedimentation of anisotropic particles in viscoelastic suspending fluids [40] , [46] . We have demonstrated enhanced inertio-elastic focusing of rigid spherical beads, deformable WBCs and anisotropic PEG particles using a common biopolymeric drag-reducing agent (HA) in a previously unexplored regime of channel Reynolds and Weissenberg numbers that can be accessed through the use of a rigid microfluidic device. We have demonstrated that there is a complex interaction between inertial effects in the flow and the viscoelastic fluid rheology that governs the migration, orientation and deformation of large (non-Brownian) particles suspended in the fluid. By varying the cross-sectional channel shape, the polymer molecular weight as well as the size and deformability of the focused particles, we have shown that it is not shear thinning or the presence of secondary flows in the channel but elastic normal stresses in the fluid that drive the strong centerline focusing behaviour observed. These discoveries will inform our future work on the design of particle sorting methods that utilize this previously unexplored flow regime. It is worth noting that the relative importance of elastic and inertial effects in the flow can be captured quantitatively by the channel elasticity number defined as El = Wi / Re as shown in Fig. 4 . The previous studies of particle migration in a viscoelastic liquid all correspond to highly elastic fluids at El >>1 (refs 16 , 17 ). In these viscoelastic fluid systems, the migration to the channel centerline increasingly worsened for channel Reynolds number exceeding Re >1, presumably due to the elastic forces on a particle being overwhelmed by the inertial forces or due to the onset of elastic flow instabilities at high Weissenberg numbers [47] , [48] . These results suggest that elastically dominated particle migration ( El >>1) toward the channel centerline should be expected to deteriorate at Re ≥ O (1), which is itself well below the threshold for inertial focusing in a microchannel [7] . However, in our study, we observe particle migration in weakly elastic fluids ( El ~0.1) toward the channel centerline over a wide range of Reynolds numbers 10≤ Re ≤10 4 , and rather than deteriorating, the focusing performance of the microfluidic device actually improves with increasing flow throughput up to Re~O (10 3 ). We show that particle migration can in fact be achieved when both elasticity and inertia are present (that is, Wi >>1 and Re >>1). Moreover, we observe controlled particle migration in a viscoelastic liquid at Reynolds numbers well beyond the upper limit previously observed for inertial focusing in a Newtonian fluid [11] . The tension along fluid streamlines resulting from weak viscoelastic effects in the fluid stabilize the flow and delay the transition to turbulence. We note that our results represent an improvement of three to four orders of magnitude in flow rate (within a single microchannel) over previous studies of particle migration in a viscoelastic fluid. With sample processing rates of up to 3 l h −1 (and linear velocities of 460 km h −1 ) in a single microchannel, and the ability to parallelize the channel design, inertio-elastic particle focusing may ultimately be used for rapid isolation of tumour cells from large volumes of bodily fluid samples (for example, peritoneal washings, bronchoalveolar lavages, urine) [49] , high-throughput intracellular delivery of macromolecules for therapeutic application [50] , scanning of multifunctional encoded particles for rapid biomolecule analysis [51] and removal of floc aggregates within water treatment systems [52] . 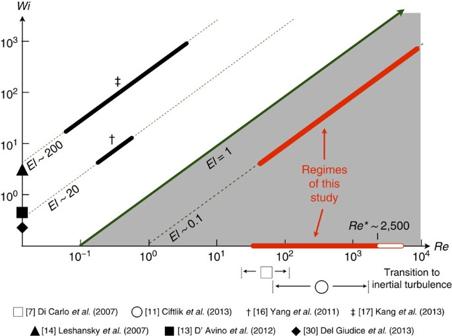Figure 4: Operating space of inertio-elastic focusing in straight microchannels. The parameter spaces probed by these studies are conveniently located on a two-dimensional plot of the fluid elasticity and the fluid inertia, as characterized by the channel Weissenberg number (Wi) and the channel Reynolds number (Re), respectively. The slope of a line passing through this space represents the value of the channel elasticity number (El); which is controlled by variations in the fluid viscosity (η), the fluid relaxation time (λ) and the microchannel dimensions. A value ofEl>1 indicates a primarily elastically dominated flow on the length scale of the channel, whereas a value ofEl<1 indicates a primarily inertially dominated flow. The red bars correspond to the range ofWiandReexplored in this study. Note that the white shaded region (beginning atRe*~2,500) within the red bar on the horizontal axis indicates the regime in which turbulent flow in the Newtonian fluid was observed. Also note that the studies of Di Carloet al.and Ciftliket al.are both in the Newtonian limit (that is,Wi=0). Figure 4: Operating space of inertio-elastic focusing in straight microchannels. The parameter spaces probed by these studies are conveniently located on a two-dimensional plot of the fluid elasticity and the fluid inertia, as characterized by the channel Weissenberg number ( Wi ) and the channel Reynolds number ( Re ), respectively. The slope of a line passing through this space represents the value of the channel elasticity number ( El ); which is controlled by variations in the fluid viscosity ( η ), the fluid relaxation time ( λ ) and the microchannel dimensions. A value of El >1 indicates a primarily elastically dominated flow on the length scale of the channel, whereas a value of El <1 indicates a primarily inertially dominated flow. The red bars correspond to the range of Wi and Re explored in this study. Note that the white shaded region (beginning at Re *~2,500) within the red bar on the horizontal axis indicates the regime in which turbulent flow in the Newtonian fluid was observed. Also note that the studies of Di Carlo et al. and Ciftlik et al. are both in the Newtonian limit (that is, Wi =0). Full size image Channel fabrication and design For the construction of epoxy devices, channel features were created using computer-aided design software (AutoCAD) and printed on a Mylar mask (FineLine Imaging). SU-8 photoresist (MicroChem) was deposited onto a silicon wafer to produce a SU-8 master consisting of straight channels ( L =35 mm) with square ( H =80±5 μm) cross-section. Polydimethylsiloxane (PDMS) elastomer (Sylgard 184, Dow Corning) was poured over the SU-8 master to generate a PDMS replica ( Supplementary Fig. 1 ). The PDMS replica was peeled off and coated with (tridecafluoro-1,1,2,2-tetrahydrooctyl)trichlorosilane (Gelest) to produce a hydrophilic surface. PDMS elastomer was poured over the silane-coated PDMS replica to generate a hydrophobic PDMS master. The PDMS master was peeled off and punched with inlet and outlet holes using a coring tool (Harris Uni-Core). One end of a 7-mm strand of 0.028" diameter Teflon cord (McMaster-Carr) was partially inserted into a 13-inch strand of PEEK tubing (Sigma-Aldrich). The other end of the Teflon cord was partially inserted into the inlet and outlet holes of the PDMS master. Epoxy resin (EpoxAcast 690, Smooth-On) was poured over the PDMS master to generate an epoxy replica. After curing, the epoxy replica was separated from the flexible PDMS master and the Teflon plugs were removed from the inlet and outlet holes. A 1-inch by 3-inch glass slide (Thermo Scientific) was coated with a 200-μm thick layer of epoxy resin. The epoxy replica and epoxy-coated glass slide were irreversibly bonded using mild (50 °C) heat from a hot plate (Thermo Scientific) and gentle pressure using tweezers (Techni-Tool). For the construction of glass devices, borosilicate glass tubing (VitroCom) with round (50-μm diameter) or square (50-μm height and width) cross-section was used. PEEK or Tygon tubing was bonded to a glass slide using an epoxy liquid (Loctite). Each end of the borosilicate glass tubing was inserted into PEEK or Tygon tubing using an epoxy gel (Loctite). The edges of the glass slide were covered with air-dry clay (Crayola), and the borosilicate glass tubing was submerged in an optically matched fluid (Sigma-Aldrich). The height H and width W of the channel cross-section were chosen to maximize the Reynolds number for a given volumetric flow rate Q and hydraulic diameter D =2 HW /( H + W ). The channel Reynolds number Re can be expressed as where ν is the kinematic viscosity of the fluid and α = H / W is the aspect ratio (with the constraint that 0≤ α ≤1). For a constant ratio of Q / D , the value of Re is maximized when α =1 ( Supplementary Fig. 6 ). The length L of the channel was chosen to ensure that the flow was hydrodynamically fully developed for all Re over which the flow was laminar. For the flow of a Newtonian fluid in a rectilinear duct [53] , the hydrodynamic entrance length L e can be expressed as with the additional condition that L e < L < L s , where L s is the length of the epoxy-coated glass slide. The transition to inertially dominated turbulence is expected to occur at Re ~2,000, which suggests that L e =113 D . For polystyrene beads with particle diameter a =8 μm, we set the hydraulic diameter D = W = H =80 μm such that the ratio of particle diameter to channel dimension a / D ≥0.1. For a straight channel with 80-μm square cross-section, we set the channel length L =35 mm, which exceeded the entrance length L e =9 mm for Re ~2,000. Sample preparation HA sodium salt (357 kDa (Lifecore Biomedical) and 1650 kDa (Sigma-Aldrich)) was added to water (Sigma-Aldrich) for bead suspensions or phosphate-buffered saline (PBS) solution (Life Technologies) solution for cell suspensions and prepared using a roller mixer (Stuart, Sigma-Aldrich). Polystyrene beads (FluoSpheres, Invitrogen or Fluoro-Max, Thermo Scientific) suspended in Tween-20 (Sigma-Aldrich) solution (0.1% v/v, water) were diluted in HA solution (1,650 kDa, 0.1% w/v, c / c *=10 (ref. 24 ), water) at a concentration of 3 × 10 6 beads per ml. WBCs were harvested from human Buffy coat samples (MGH Blood Bank) via density gradient centrifugation (Histopaque-1077, Sigma-Aldrich). WBCs were centrifuged and suspended in Calcein Red-Orange solution (10 μg ml −1 , PBS). Fluorescently labelled WBCs were centrifuged and suspended in PBS, low-molecular weight HA solution (357 kDa, 0.1% w/v, PBS) or high-molecular weight HA solution (1,650 kDa, 0.1% w/v, PBS) at a concentration of 5 × 10 6 cells ml −1 . Anisotropic (cylindrical) hydrogel particles were synthesized via stop-flow lithography [45] from prepolymer solutions of 60% poly(ethylene glycol) diacrylate (PEG-DA 700, Sigma-Aldrich), 30% poly(ethylene glycol) (PEG 200, Sigma-Aldrich), 10% 2-hydroxy-2-methylpropiophenone (Sigma-Aldrich), and 3 mg ml −1 rhodamine acrylate (Polysciences). Fluorescently labelled PEG particles (20-μm length, 10-μm cross-sectional diameter) were collected and washed in Tween-20 solution (0.1% v/v, PBS) before dilution in HA solution (1,650 kDa, 0.1% w/v, water). Microparticles suspended in Newtonian or viscoelastic fluids were prepared in 100-ml volumes to maximize observation time of particle flow, especially at the upper limit of flow rates in the rigid microchannel. Fluid rheology measurements The viscosity of all fluid samples was measured using both a stress-controlled rheometer (DHR-3, TA Instruments) and a microfluidic viscometer-rheometer-on-a-chip (VROC, Rheosense) ( Supplementary Fig. 3 ). The DHR-3 instrument imposed an increasing shear rate ramp on a fluid sample contained within a double-gap cylindrical Couette cell. The viscosity of the fluid sample was measured on the DHR-3 instrument for shear rates . The VROC microfluidic chip consists of a borosilicate glass microchannel with a rectangular slit cross-section and a silicon pressure sensor array. The viscosity of the fluid sample was measured on the VROC device for shear rates . In order to numerically predict the velocity profiles in the channel, the measured flow curve of the native sample was fit with the Carreau model where η ∞ is the infinite-shear rate viscosity, η 0 is the zero-shear rate viscosity, is a characteristic shear rate at the onset of shear thinning, and n is the ‘power-law exponent’. We measured the fluid viscosity of both native and used samples of HA solution at Q =20 ml min −1 to investigate the role of shear-induced sample degradation. The viscosity of native HA solution exceeded the viscosity of used HA solution by at least a factor of 2 for shear rates presumably due to the shear-induced disruption of aggregates in the solution. However, the measured difference in HA viscosity between the samples was minimal and remained unchanged after repeated shearing for the high shear rates ( ) explored in this study. This suggests that irreversible polymer degradation had little to no effect on HA viscosity at the flow rates where particle focusing was observed. The relaxation time λ of the native HA solution was measured based on thinning dynamics in jetting experiments [25] . As a viscoelastic liquid bridge thins, the diameter of the filament D will decay according to the relation [54] where D o is the initial diameter of the filament. When plotted on semi-logarithmic axes, the initial slope of filament decay is equal to −1/3 λ ( Supplementary Fig. 7 ). Pressure drop measurements Fluid flow through the microchannel was achieved using a syringe pump (100DX, Teledyne Isco) capable of a maximum flow rate of 50 ml min −1 , a maximum pressure of 10,000 psi and a maximum capacity of 103 ml. A stainless steel ferrule adapter (Swagelok) connected the syringe pump to the PEEK tubing embedded in the epoxy chip. The syringe pump’s internal pressure transducer was used to obtain pressure drop measurements across the entire fluidic circuit. However, we found that the hydrodynamic resistance of the microchannel accounted for approximately 99% of the overall hydrodynamic resistance. As a result, we considered the pressure drop measured by the syringe pump to be essentially equal to the pressure drop along the microchannel. The pressure drop Δ P was an essential parameter in determining the friction factor f , defined for laminar flow of a Newtonian fluid through a square microchannel as where U is the mean fluid velocity in the channel, L is the channel length, D is the channel hydraulic diameter and Re is the channel Reynolds number. In this operating regime, Δ P increased linearly with Q , and f scaled inversely with Re . For Re >2,000 (where the channel flow is expected to be turbulent), f can be expressed in a microchannel [55] as where ε = k / D is the ratio of the average surface roughness on the channel wall k to the channel hydraulic diameter D . The typical surface roughness was k ~ O (1 μm) for the epoxy channels used in this study. As a conservative estimate, we set ε ~0.01 to calculate f as a function of Re . The characteristic viscosity was an essential parameter for determining the channel Reynolds number, and the Carreau model was used to calculate the characteristic viscosity as a function of wall shear rate. For Newtonian flow in a square microchannel (that is, α =1), the analytical solution [55] of wall shear rate can be expressed as When the characteristic viscosity (based on wall shear rate) is used to calculate Re , the friction factor of the HA solution f HA collapses onto the expected curve for a Newtonian fluid ( Supplementary Fig. 8 ). Velocimetry measurements Images of fluorescent particles in the microchannel were acquired with a Nd:YAG dual cavity 90 mJ per pulse laser (LaVision) that was frequency doubled to emit green light at 532 nm, a 1.4-megapixel CCD camera (PIV-Cam 14-10, TSI) and an epifluorescence microscope (TE-2000, Nikon). The pulse width for the laser was approximately δ t ~10 ns, yielding an instantaneous power that was approximately 90 MW. The fluorescent signal from the particles is passed through a barrier filter and dichroic mirror [56] . This allows for the elastically scattered light from the illumination source (532 nm laser) to be filtered out while leaving the fluorescent emission (at a longer wavelength) to pass through to the CCD camera virtually unattenuated [57] . The minimum time between consecutive laser pulses was Δ t interpulse,min ~200 ns, and the minimum interframe time (that is, time between consecutive images) was Δ t interframe ~1.2 μs. For a given flow rate, the time interval between the two consecutive laser pulses was user defined to achieve a maximum particle displacement of approximately eight pixels (which is the optimal displacement for the correlative PIV algorithm used in this study). For Q <0.1 ml min −1 , the time required between laser pulses (Δ t interpulse ) to achieve this optimal displacement was greater than the camera interframe time (Δ t interpulse >Δ t interframe ), which enabled observation of particle displacement over two single-exposed images. Therefore, at these low flow rates, the PIV analysis was completed in frame straddling mode, which relies on a cross-correlation approach between the image pair [58] (TSI). Conversely for Q >0.1 ml min −1 , the time step required for optimal particle displacement was less than the interframe time (Δ t interpulse <Δ t interframe ), and particle displacement was observed over one double-exposed image. Hence, at these higher flow rates, the PIV analysis was done using an auto-correlation approach (LaVision). Particle velocity measurements were made with 8-μm polystyrene beads (3 × 10 6 beads per ml water or HA solution), and fluid velocity measurements were made with 1-μm polystyrene beads (3 × 10 8 beads per ml water or HA solution). At a given x–z plane, microparticle image velocimetry was used to record the displacement of 1-μm beads within an array of interrogation windows over a given time interval. At the same x–z plane, PTV was used to record the displacement of 8-μm beads in the x -direction over a given time interval ( Supplementary Fig. 9 ). PTV images were processed in MATLAB (MathWorks) to generate a set of individual particle velocity measurements. It is worth noting that some particle blurring in the fluorescent images can occur at the highest flow rates explored in this study, even with an extremely short pulse duration of δ t ~10 ns. For the microscope objective and camera used in this work, one pixel corresponds to ( eM ) 2 =0.323 × 0.323 μm 2 , hence the fluid velocity necessary for a particle to traverse one pixel during a single laser pulse (and thus show blurring) is U blur ~( eM )δ t −1 =32 m s −1 which corresponds to the maximum fluid velocity for Q ≈6 ml min −1 ( Fig. 2c ). For the 1-μm particles that were used to measure the fluid velocity profile, a blur length of one pixel is a significant fraction of the particle diameter, which can adversely affect the accuracy of the correlative PIV algorithm [59] . For this reason, quantitative velocity profile measurements were not performed at higher flow rates where the blurring would be severe. In a typical velocimetry measurement, a 1-μm tracer particle travels approximately four to eight pixels between consecutive laser pulses, which corresponds to a 13% to 25% error. On the other hand, a typical 8-μm particle used in this study has a diameter of around 25 pixels in a single microscope image, hence even at the highest velocities considered in this study around U =130 m s −1 ( Q =50 ml min −1 ), the expected blurring will be approximately four pixels, which is only 16% of the particle size. How to cite this article: Lim, E. J. et al. Inertio-elastic focusing of bioparticles in microchannels at high throughput. Nat. Commun. 5:4120 doi: 10.1038/ncomms5120 (2014).